Similarities between protein folding and granular jamming Granular matter (such as sand, coal or powder) is rigid when jammed, but flows when external loads are applied. Experiments show that jammed grains resist flow by forces that are propagated through the material across percolating networks of immovable particles, complex sets of force chains that give rise to rich phenomenology [1] , [2] . Different in nature from grains, glasses, obtained from supercooled liquids that avoid crystalization [3] , are also rigid when cold, but flow when their temperature is increased. Grains and glasses seem to ‘unjam’ alike; the physical change they have in common is a variation in their mechanical response to external perturbations from a stable, disordered configuration to a flowing, loose state. Common behaviour has been suggested to exist in the form of a ‘universal jamming phase diagram’ [4] mapping the arrest of dynamics in all such systems (see Fig. 1a ). This commonality is despite the fundamentally distinct nature of the interactions involved: for glasses, which are atomic systems, the inter-particle energies are comparable to k B T and unjamming occurs due to thermal effects, whereas granular matter belongs to a completely different class. The characteristic interactions between grains are so large that temperature is irrelevant and energy dissipates almost instantaneously through friction (making difficult—except for simple models [5] —a traditional statistical mechanical approach). For the athermal grains, unjamming occurs because of the external field applied. In the wake of the conjecture of the universality of the jamming diagram, phenomenology common to jammed grains [6] and supercooled systems has been sought and reported increasingly frequently [5] , [7] , [8] , [9] , [10] , [11] , [12] , [13] , in an effort to unify glass and jamming transitions. However, a common theory for the origins of the assumed unification is lacking, chiefly because the interactions responsible for the dynamical arrest are so different. More importantly, detailed new experiments on grains have revealed that there are differences even within the granular realm itself; under a variety of conditions, a more complex picture of jamming than that sketched in the original jamming diagram is emerging. This includes the intricacies of the preparation protocol, which can induce granular jamming into several distinct states [14] , a more subtle role of shear than originally envisaged [15] , [16] , [17] , and the importance of frictional interactions [18] . A more complex jamming scenario, rather than a single, overarching universality, is also revealed when considering criticality arguments; upon approaching a critical value Φ c of the jamming order parameter Φ (for example, the packing density), zero temperature granular matter develops correlations that diverge like | Φ − Φ c | −γ (refs 19 , 20 ). But unlike universal power law divergence around thermodynamical critical points, in granular matter, depending on the shearing conditions, different groups (working on different systems and/or conditions) find different critical exponents γ (refs 21 , 22 , 23 ). 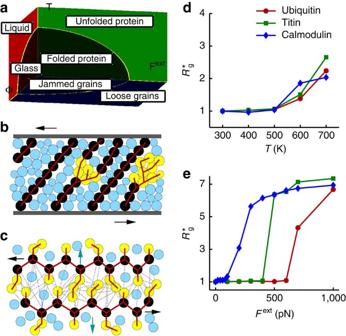Figure 1: Parallels between jamming and folding transitions. (a) Schematic phase diagram for ‘unified jamming’ adapted from ref.4to proteins. Below certain values of external force (Fext), temperature (T) and denaturant concentration (Φ, or other environmental parameter), proteins fold and undergo changes in mechanical properties similar to jamming of grains. (b,c) Caricatural analogy between shearing jammed grains and unfolding proteins: (b) jammed grains: black beads carry stress balancing paths, yellow depicts less stress bearing beads, and blue beads are least stressed, loose grains (cf. Cateset al.2). Force chains marked with red lines; black arrows indicate direction of shear. (c) Proteins pulled by external forces (in analogy with panelb), with backbone as the force transmission path (colour coding of atoms-beads correspondence as inb); the dotted lines depict non-bonding interactions. (d,e) Radius of gyrationRg*=Rg/Rg|T=300K,Fext=OpNof proteins versusTandFext; a sudden increase ofRgdefines the transition values ofTandFextwhere proteins loose majority of native contacts and ‘unjam’. Figure 1: Parallels between jamming and folding transitions. ( a ) Schematic phase diagram for ‘unified jamming’ adapted from ref. 4 to proteins. Below certain values of external force ( F ext ), temperature ( T ) and denaturant concentration ( Φ , or other environmental parameter), proteins fold and undergo changes in mechanical properties similar to jamming of grains. ( b , c ) Caricatural analogy between shearing jammed grains and unfolding proteins: ( b ) jammed grains: black beads carry stress balancing paths, yellow depicts less stress bearing beads, and blue beads are least stressed, loose grains (cf. Cates et al. [2] ). Force chains marked with red lines; black arrows indicate direction of shear. ( c ) Proteins pulled by external forces (in analogy with panel b ), with backbone as the force transmission path (colour coding of atoms-beads correspondence as in b ); the dotted lines depict non-bonding interactions. ( d , e ) Radius of gyration R g * = R g / R g | T =300 K , F ext =OpN of proteins versus T and F ext ; a sudden increase of R g defines the transition values of T and F ext where proteins loose majority of native contacts and ‘unjam’. Full size image Important clues have emerged from experiments on grains and colloids, and from simulations of glasses. For grains approaching jamming, a signature of the transition develops in the form of a measurable peak in the low-force region of the distribution of contact force components [24] , [25] , [26] , [16] , a peak non-existent in the loose, unjammed state. Simulations of grains as frictionless particles confirmed the onset of such a peak on jamming [27] . In the realm of glasses, atomistic simulations of glass-forming liquids also have shown that a peak appears in the inter-particle normal force near [7] , [9] or, in one case, much below [8] the glass transition temperature T g and have suggested that the peak is related to the fragility [3] of the glass former. On the other hand, in the realm of grains, ‘fragility’ refers to states that are robust under continued shear, but that unjam if the shear changes direction. This fragile response was linked [2] to the marginal stability of the percolating network of force chains [1] within the material (see Fig. 1b ). Concomitant with results on several granular systems for which a peak in the force distribution was deemed symptomatic of jamming, important subtleties have been observed. The force distribution can have a more complex connection to the state of the system. For example, the shape of the peak for jammed systems is sensitive to whether the system is sheared (that is, if external load is anisotropic) or not [15] , [16] , [28] . At the same time, the long f -tails are functionally sensitive to external stress conditions (see below). Although a jamming peak appears in both grains and glasses, temperature-controlled and load-controlled jamming are usually observed in different systems, because it is difficult to apply forces to temperature-dependent glasses and it is difficult to define a temperature for grains under load. Therefore, with a few notable exceptions, such as a study of attractive colloids under external stress [6] and the rheology of vibrated disks [29] , [30] (which however—even when the vibration balances dissipation—are in non-equilibrium steady states at best, and do not truly reach thermal equilibrium, but thermodynamic analogies of which are nonetheless intriguing [31] ), systems for which jamming occurs collectively across the T − F ext plane ( Fig. 1a ) are scarce, because when acting naturally F ext and T are applied in different systems (throughout the paper, we denote by F ext the external force applied on the system to distinguish it from internal forces F on each particle). Here we suggest that proteins are systems that naturally populate the T − F ext plane and aim to describe their folded states using the language and descriptors of jamming. In the process, we reveal parallels, but also differences, between the protein-folding transition and the jamming transition. The study is of relevance, because proteins are systems whose dynamics and thermodynamics are naturally modulated by both the temperature and external force. First, increasing temperature above a certain folding temperature induces reversible protein unfolding [32] ; this temperature-controlled change is akin to a glass-to-liquid transition. As such, rich theoretical advancement has been made for protein folding using an energy landscape description inspired by glasses [33] , [34] . Second, many proteins, such as those translocated through membranes or those degraded by ATP-dependent proteases, undergo regulated unfolding in vivo under the influence of externally applied forces [35] . Proteins are also unfolded in vitro by single-molecule pulling with atomic force microscopy, optical or magnetical tweezers to study the heterogeneity of their unfolding pathways [36] ; under such external loads, signatures of glassy dynamics are again manifested [37] . Temperature and force unfolding of proteins We chose proteins calmodulin, titin (the I27 module) and ubiquitin from the three major types of secondary structure combinations: all α-helical, all β-sheet and mixed, respectively. The three proteins were simulated using molecular dynamics simulations [38] in their native, folded states, as well as at increasing temperatures, T , or under increasing external forces, F ext , applied at the two ends (all at T =300 K) to induce protein unfolding. We used the variation of their radius of gyration R g as a gauge of the degree of protein unfolding ( Fig. 1d ). Samples from the various temperature- and force-dependent molecular dynamics trajectories were used to generate structural ensembles of folded or unfolded structures (depending on the value of T or F ext ). With these ensembles, we then set to explore how variations in the interatomic force distributions correlate with the folding–unfolding transition. Moreover, proteins are macromolecules with a well-defined connectivity along the bonded backbone, which can act, on the application of external forces, as stress transmission paths that are heuristically comparable to force chains in granular materials (compare Fig. 1b with c ). As in any given protein the same interactions are responsible for both the temperature- and force-induced unjamming, we set to directly compare which protein microscopic signatures may, at the onset of jamming, be common with granular-like and glass-like matter. Given that in their thermal unfolding proteins contain vestiges of the glass-to-liquid (that is, unjamming) transition, it is tempting to regard protein unfolding by external pulling at their ends in similarity to unjamming grains by external shear force. However, complexities arise. Stress chains fail in sheared dry non-cohesive granular material because of compression in the chain direction and by a process akin to buckling. The physics of buckling under compression and that of failure by extension, the later being the process for the present study, are generally not the same. In the case of proteins, unjamming under extension may correspond to a different failure mode. The analogue of the pulling scenario for a granular system would require cohesive grains (cf. Fig. 1b ), and such a system might have a different phenomenology worth testing in its own right, for example, in attractive colloidal suspensions [6] (also, see below the discussion on force pulling). We note that graphs like the schematic universal phase diagram were produced as a result of using lattice and off-lattice models to understand the collective effect of external force and temperature, and temperature softening and related ideas were discussed (see refs 39 , 40 ). Signatures in the distribution of forces Using ingenious measurements, experiments on jammed grains [41] and colloids [42] have recorded entire distributions of single-particle forces, which reveal a peak upon jamming as discussed. To compare with these experimental data, we have computed from our simulations F =|−∂ V /∂ r i |, ∀ i , that is, the force magnitude on any single particle i due to all terms in the potential energy function V ({ r i }). We then normalized forces in all cases (simulation and experiment) by f = F /〈 F 〉, with 〈 F 〉 the average force over all force data for the corresponding system (proteins, grains, colloids). Despite the span of nine orders of magnitude between atomic and grain forces, an absolutely remarkable universal peak ( Fig. 2 ) became apparent in all the distributions P ( f ) of scaled forces for grains, colloids and the three proteins. 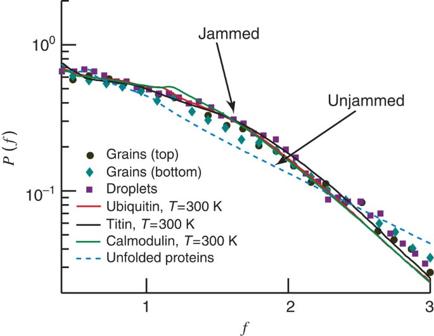Figure 2: Universal shape of the jamming peak. The shape of the distributionsP(f) of scaled forcesf=F/〈F〉 for protein atoms (from our simulations of the folded states), jammed grains (from experimental data reported in ref.41) and jammed droplets (from experimental data in ref.42) fall on a universal curve. Figure 2: Universal shape of the jamming peak. The shape of the distributions P ( f ) of scaled forces f = F /〈 F 〉 for protein atoms (from our simulations of the folded states), jammed grains (from experimental data reported in ref. 41 ) and jammed droplets (from experimental data in ref. 42 ) fall on a universal curve. Full size image To directly compare with structural signatures of jammed glasses [7] , whose atomic interactions have an important long-range component, we have computed the non-bonded contribution to the force distribution, P nb ( f nb ), where the scaled forces were f nb = F nb /〈 F nb 〉, with , being the magnitude of the force on any atom i from non-bonded pair interactions (electrostatic and van der Waals) with all the other atoms j . In Fig. 3 , the distribution P nb ( f nb ) also shows a peak when the proteins are folded, as already shown for P ( f ). As for P ( f ), the height of the peak in P nb ( f nb ) decreases as T or F ext increase; this reflects a decrease in the degree of jamming. Unlike the universal peak in P ( f ), however, the size of the peak in P nb ( f nb ) is protein-dependent, being more pronounced for more mechanically stable proteins. For the curves plotted in Fig. 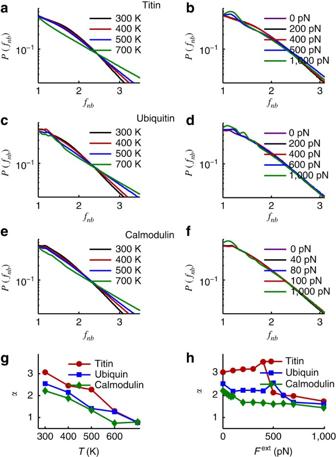Figure 3: Temperature- versus force-induced unjamming. Peak disappearance upon temperature and force unfolding for the three proteins studied. Semi-log plot of force distributionPnb(fnb) for non-bonding interactions against scaled forcefnb. Variation ofPnb(fnb) under differentTs shown ina,c,e, and under differentFextinb,d,ffor titin (a,b), ubiquitin (c,d) and calmodulin (e,f). For highFextforces (that is, beyond unfolding, for example, green curve inFig. 3b), note the additional ‘ripples’ appearing for smallfnbin accord with data on triangular lattices under increasing anisotropy of shear (cf., for example,Fig. 5in ref.46and references therein). Variation of exponentα(a measure of peak size) againstTin panelg, andαagainstFextinh. The magnitude ofα(see text) correlates with the mechanical unfolding resilience and may be considered as a measure of the amount of stress stored in the non-bonding interactions. Titin, which has highest value ofα, is one of the strongest proteins found in nature. 3 , the dependence P nb ( f nb ) around the peak can be fitted to a function of the form Figure 3: Temperature- versus force-induced unjamming. Peak disappearance upon temperature and force unfolding for the three proteins studied. Semi-log plot of force distribution P nb ( f nb ) for non-bonding interactions against scaled force f nb . Variation of P nb ( f nb ) under different T s shown in a , c , e , and under different F ext in b , d , f for titin ( a , b ), ubiquitin ( c , d ) and calmodulin ( e , f ). For high F ext forces (that is, beyond unfolding, for example, green curve in Fig. 3b ), note the additional ‘ripples’ appearing for small f nb in accord with data on triangular lattices under increasing anisotropy of shear (cf., for example, Fig. 5 in ref. 46 and references therein). Variation of exponent α (a measure of peak size) against T in panel g , and α against F ext in h . The magnitude of α (see text) correlates with the mechanical unfolding resilience and may be considered as a measure of the amount of stress stored in the non-bonding interactions. Titin, which has highest value of α , is one of the strongest proteins found in nature. Full size image with f 0 and A constants, and the fitting parameter α >1 giving a measure of peak size. The variation of α correlates with the perception of mechanical resilience to unfolding. Values of α close to unity (that is, no peak) are seen in the unjammed states, whereas the maximum value of α (largest peak) corresponds to the maximally jammed state (that is, at null F ext and room temperature) of the maximally stable protein. Figure 3g ranks titin highest in stability, stability that decreases as T increases; ubiquitin is next and calmodulin is least stable; the same order of mechanical resilience was found in the single molecule pulling experiments [43] , [44] , [45] . Figure 3h shows that this α -ordering holds for our force-dependent unfolding data, too; under F ext , α is a measure of the increase of jamming. Near the sudden break of the folded structure, α decreases for small increments of F ext . On further increases of F ext , unfolding (that is, the jamming to unjamming transition) ensues. Our results suggest that an analysis of P nb ( f nb ) in the folded state of a wide range of proteins, with a tabulation of the respective α -values, may have predictive power in ranking mechanical or thermal stability. Moreover, it is known that, depending on the protocol for minimization during, for example, simulated annealing, proteins can be trapped in metastable states around the folded state. This is also analogous to the dependence of the glass transition temperature on the cooling rate in glasses. We expect that the distributions P nb ( f nb ) of trapped intermediates can feature peaks similar to the folded state, but with α -values correlating to stability. Jamming in frictionless granular systems also can feature a multiplicity of jammed states surrounding the frictionless point in the phase diagram [14] , accessing each requiring a different preparation protocol. An analogy to such protocol-dependent, distinct jammed states might be present in studies of metastable conformational states in proteins. Although the peak fits the super-exponential form in equation 1, that is, with α >1) in the low-force region (around f≈ 1), the force distribution of the pair forces P nb ( f nb ) at the high-force end shows a stretched exponential tail, , with β <1 in the folded state. Analysis of individual-type interaction (that is, of each interaction between the same pair type of atoms i and j ) revealed an exponential pair-force distribution tail (in accord with the simulations of Lennard–Jones systems) and differences in the peak shape and position (see Supplementary Fig. S1 ). The decay constant f 0 of each of the tails for different atom pairs are however different; thus, their superposition leads to a stretched exponential. Upon unfolding, β →1 because a limited number of interaction types exists within the non-bonded cut-off and through the backbone in the unfolded state; this narrows considerably the distribution of characteristic decay forces extant in the folded state and stretched exponentiality hence subsides. Comparison of pairwise unscaled force distributions P ( F ij ) in equilibrium with thermally and force-unfolded states ( Fig. 4a ), respectively, shows that the peak centres ∼ 5–15 pN in the folded state and that it disappears in both scenarios of unfolding. Note (cf. inset to Fig. 4a ) that the protein peak is the region where contributions from the bonding and non-bonding components of P ( F ij ) are comparable (bonding interactions dominate P ( F ij ) in the high-force end, whereas the non-bonding interactions dominate in the low-force region). On the other hand, there is no peak disappearing in the bonding distribution upon either T - or F ext -unjamming. This indicates that the peak arises from the non-bonding interactions that are transmitted through the bonded structure (the skeleton) of the protein, that serves as a force chain for jamming. We also note, making again reference to the inset of Fig. 4a , that, over the low-force region, P ( F ij ) is scale-free for non-bonding interactions, decaying as a power law . Interestingly, the value of γ is the same; it approximates 1.6 for all three proteins in the folded state studied herein and 1.5 in the unfolded state in all trajectories. 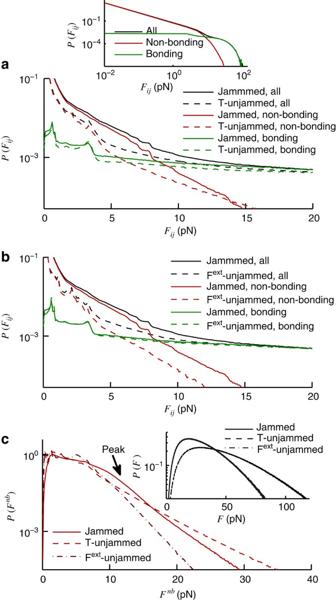Figure 4: Non-bonding contributions to the force peak. (a) Pair-force distributionP(Fij) for ubiquitin for bonding, non-bonding and all-type interactions are compared between two states: equilibrium folded state at 300 K (jammed) and thermally unfolded state atT=700 K (T-unjammed). Probability density between 5 and 15 pN, (that is, the peak) disappears upon both force- and temperature-induced unfolding for non-bonding forces only. Inset ofashows log–log plot ofP(Fij) for the full range of forces; non-bonding interactions prevail in the low-force region and bonding interactions prevail at the high-force end. (b) Comparison ofP(Fij) for folded state at 300 K without external force (jammed) and force-unfolded state atFext=1,000 pN (Fext-unjammed). (c) The distributionP(Fnb) of total non-bonded force on each atom is compared for: jammed (folded) state at 300 K, thermally unjammed atT=700 K and unjammed under external forceFext=1,000 pN. Inset ofcshows corresponding force distribution of total force on each atom from all contributions (bonding and non-bonding) over the entire force range. Figure 4: Non-bonding contributions to the force peak. ( a ) Pair-force distribution P ( F ij ) for ubiquitin for bonding, non-bonding and all-type interactions are compared between two states: equilibrium folded state at 300 K (jammed) and thermally unfolded state at T =700 K ( T -unjammed). Probability density between 5 and 15 pN, (that is, the peak) disappears upon both force- and temperature-induced unfolding for non-bonding forces only. Inset of a shows log–log plot of P ( F ij ) for the full range of forces; non-bonding interactions prevail in the low-force region and bonding interactions prevail at the high-force end. ( b ) Comparison of P ( F ij ) for folded state at 300 K without external force (jammed) and force-unfolded state at F ext =1,000 pN ( F ext -unjammed). ( c ) The distribution P ( F nb ) of total non-bonded force on each atom is compared for: jammed (folded) state at 300 K, thermally unjammed at T =700 K and unjammed under external force F ext =1,000 pN. Inset of c shows corresponding force distribution of total force on each atom from all contributions (bonding and non-bonding) over the entire force range. Full size image Showcasing ubiquitin as an example (titin and calmodulin show similar profiles and characteristic peak forces (see Supplementary Fig. S2 ), Fig. 4c shows that the force distribution of the sum of the forces on each atom from non-bonding interactions P ( F nb ) also develops a peak for the folded state relative to the distributions recorded upon thermal or force-induced unfolding. The inset to Fig. 4c shows the distribution P ( F ) of the total forces on each atom from all contributions (bonding and non-bonding) over the entire spread of forces in the folded versus unfolded state. Comparison of Fig. 4c with its inset shows that, when the protein unfolds the non-bonding force distribution contracts, whereas the all-type contribution (that is, from bonding plus non-bonding forces) spreads; this is attributed to the fact that when the protein is unfolded, stress relaxation through non-bonding interactions reduces. In the inset ( Fig. 4c ), the all-type distribution P ( F ) for unjamming under a force so high that it pulls the protein taut ( F ext =1,000 pN) coincides with the T =300 K jammed (folded) state. This is because in the distribution P ( F ) of the total forces F , the major contribution is from bonding interactions (contribution from non-bonding interactions are negligible). The force distribution of the bonding interaction varies significantly only with temperature variation; it shows negligible changes upon force unjamming at the same temperature. So taken together, where do our results on protein force distributions stand in relationship to the universal jamming diagram? Is protein folding in a universality class with grains, glasses and other systems undergoing dynamical arrest? The answer is complex. The conjecture by O’Hern et al. [7] has put forth that the peak in P ( f ) is symptomatic of jamming. Our results herein also show that a peak appears in folded proteins. However, even for grains, several subtleties have been revealed regarding the overall shape of P ( f ) (that is, peak and tail) and its relation to jamming. Evidence is accumulating from several granular studies that both the peak shape and the large f -tail of the distribution are strongly influenced by anisotropy, not just by (un)jamming. The effect of anisotropy on the peak was explored theoretically [15] , [28] (see also review by Tighe et al. [46] ). For small f , rippling in P ( f ) has been shown in frictionless triangular lattices under increasingly anisotropic external shear stress (compare, for example, Fig. 5 in ref. 46 with ripples for high F ext , for example, green curves in our Fig. 3b ). Experimentally also, the peak was shown to be different in purely sheared versus uniformly compressed grains [16] . The same experiments also revealed changes in the tail of P ( f ), with theory [46] showing an exponential character in the tails evolving as the shear stress/normal stress grows. This leaves the exact shape of P ( f ) still an open question for granular materials, and this richness in details is reflected by our results in the protein realm. 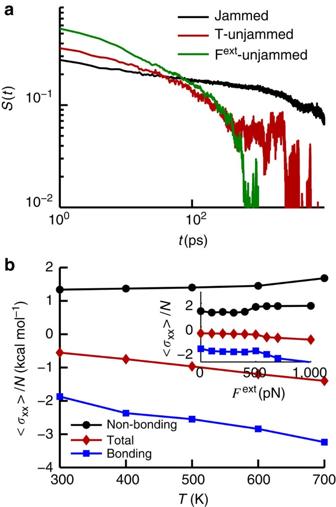Figure 5: Stress relaxation as a dynamical signature of jamming. (a) Normal stress–stress correlation functionS(t) for folded, thermally unfolded and force-unfolded states for titin from equilibrium trajectories. (b) Dependence of average stress 〈σxx〉/Nat different state points with increasing temperatureTand, in inset, external forceFext. Figure 5: Stress relaxation as a dynamical signature of jamming. ( a ) Normal stress–stress correlation function S ( t ) for folded, thermally unfolded and force-unfolded states for titin from equilibrium trajectories. ( b ) Dependence of average stress 〈 σ xx 〉/ N at different state points with increasing temperature T and, in inset, external force F ext . Full size image Time-dependence of stress relaxation Another characteristic property of jammed granular matter is the slowing down of stress relaxation [47] , [48] , a dynamic signature resembling the viscous slowdown of glasses [3] . Given the commonality of the jamming peak in the force distributions across folded proteins, grains and glasses, we expected that whenever jamming in the conventional sense occurs in a protein (that is, when folding occurs) stress relaxation throughout the protein should also slow down, relative to the unfolded state. To report on the mechanical stress at the atomic scale, we used the internal virial stress tensor , where μ and ν label the Cartesian components x , y , z of the position and particle force vectors, respectively, and the summation is the overall atoms. We also computed the non-bonded contribution to the virial, , with and being the ν and μ components of the non-bonding pair force and distance, respectively, between two atoms i and j . We gauged stress relaxation by the decay of the normalized stress–stress time correlation function S ( t )=( C ( t )− C (∞))/( C (0)− C (∞)), where C ( t )=〈 σ μν ( t ) σ μν (0)〉. The correlations S ( t ) in all directions did slow down in the folded state versus the unfolded ones. For example, Fig. 4a shows the decay of the S ( t ) component μ = ν = x , with the x axis alligned in the direction connecting the carboxy and amino termini (which was also the direction of pull for cases when F ext was applied). Within the folded state and in the absence of temperature increases or applied forces, S ( t ) decays slowly as a power law in time; the native contacts provide the protein with the ability to store stress. Upon moderate heating or under low external forces, such that folding is maintained, relaxation is still slow, similar to that in the absence of heating or pulling. However, for temperatures T and external forces F ext large enough to induce unfolding, the system exhibits a significantly faster, exponential tail ( Fig. 5a ). Hence, when the native contacts are maintained, the slow, power law stress–stress time correlation decay accompanies the presence of force peaks in P ( f ) and P nb ( f nb ). We also explored how the average stress itself varies as a function of the increase in T and F ext ; this would measure the change in the mechanical response of the proteins as native contacts are disrupted. To this end, we computed the particle-normalized average stress 〈 σ xx 〉/ N (angle brackets denote time averaging) and its components, the bonded and non-bonded contributions to the stress virial ( Fig. 4b ). Although the total average of 〈 σ xx 〉/ N varied as − k B T , in accord with the generalized equipartition theorem, the bonded and non-bonded terms have opposite signs (cf. Fig. 5b ). This implies that there is mutual frustration between bonding and non-bonding interactions; on the average, conformations inside a confining basin minima of the bonding potential energy are on barrier tops (destabilizing, non-minima) of the non-bonding potential. The fact that frustration increases only slightly, if ever, upon unfolding (cf. Fig. 5b and its inset) is consistent with the minimal frustration principle [49] , which states that naturally occurring proteins have evolutionarily designed sequences that fold efficiently to an ensemble of structures with hardly any traps arising from mismatch between energetic contributions. It will be of interest to analyse force and virial stress distributions, and relaxation in native sequences versus decoy proteins [50] comparatively for a microscopic description of frustration. In summary, how akin are folded proteins to jammed grains? Our simulations of force distributions and the time scales for dynamical slowdown of stress relaxation for folded versus unfolded proteins indicate several similarities, when comparisons are made with the corresponding measures in the granular states. However, a more varied connection between these measures and structural or external properties as described above for grains point to a more nuanced picture. Lessons learned from the complexities of granular jamming warrant further investigations in proteins, particularly as interactions in proteins are more complex, of multiple types, and on multiple length and time scales. For example, mechanical response in jammed granular matter is fundamentally different from that of ordinary solids. Jammed grains can make ‘fragile’ materials [2] that may jam or unjam, depending on the direction of the applied forces. Proteins seem to share such unusual mechanical properties in the sense that an individual protein exhibits different resilience to unfolding under external pulling with atomic force microscopy or single-molecule tweezers, depending on the direction of the pull [44] , [51] . Novel lock-in force spectroscopies with improved resolution [52] can directly observe reversible folding–refolding events and have even been used to measure the distributions of refolding forces at various temperatures [53] . Repeated on circular permutants (same sequence and fold, but different termini), they may be used to directly probe equilibrium forces on different protein atoms in further testing of the jamming signatures found in our study. Fragility may also be linked with the criteria for brittle response as quantified by Hyeon and Thirumalai [54] ; a protein is brittle or soft depending on the displacement of the free-energy barrier along the unfolding reaction coordinate as a result of the application of external forces. As such, it will be of interest to study the correlation between the external force-induced change in shape of the jamming peaks of P ( F ) and the change in free-energy profiles along different unfolding directions. More generally, approaches presented herein may be used to develop techniques borrowed from soft matter theory to characterize protein folding as induced self-organization of stress-propagating paths or force chains across the protein tertiary structure. Studying proteins with jamming measures may be important in the design of biomimetic polymers with responses to external mechanical stress that can be modulated by optical or thermal means, or controlled depending on the direction of stress application. Results derived herein suggest a route to designing novel resilient materials via an optimization of particle composition to yield specific interactions that augment the peak in the force distribution, or to rank the mechanical strength across various material compositions depending on the value of α . Gauging force distributions and stress relaxation may shed light in cases where proteins can jam during their response to external forces as part of their function in vivo ; for example, in muscles, in the cytoskeleton, or on passage through cellular pores. Computational details The initial co-ordinates for the simulations were crystal structures of ubiquitin (PDB id 1UBQ [55] ), titin (1TIT [56] ) and calmodulin (1LJK [57] ) obtained from the Protein Data Bank. Molecular dynamics simulations were performed by 1 fs time-step integration of Langevin dynamics with a friction co-efficient of 10 ps −1 using the CHARMM [38] software package with a united-atom force field and the analytical continuum electrostatics [58] implicit solvent model. In separate simulations, the three protein structures were equilibrated and run at T =300 K, then independent equilibration and production was repeated at increasing temperatures in the 300–700 K interval in steps of 100 K, to induce complete protein unfolding. The variation of their radius of gyration R g measured the degree of protein unfolding as shown Fig. 1d . Similarly, external forces F ext of increasing magnitude were applied at the two ends (all at T =300 K) up to 1,000 pN in steps of 100 pN. The R g variation under F ext for the three proteins is recorded in Fig. 1e . For a trajectory cut-off time of 100 ns, ubiquitin was stable until T =600 K . Under F ext at 300 K (20 ns), it unfolded above forces of 600 pN. For the same cut-offs, the corresponding values of titin are 600 K and 500 pN. Calmodulin, which has less mechanical strength, unfolded in our simulations at 400 K and at pulling forces above 200 pN. Note that these transition values are simply those at which unfolding is induced on the relatively fast time scale of the simulations, and are not supposed to directly match those measured in bulk experiments of stability. For all T -dependent studies, simulations were 100 ns long. The non-equilibrium pulling simulations were performed with constant tension F ext applied at the ends of the protein until unfolding occured (typical times ranged from 10 to 100 ns). For all simulations where unfolding occurred, only the equilibrated unfolded structures were recorded and included in the force distribution, the average stress and the stress–stress correlation analysis. The stress was measured along a fixed axis in the protein to avoid global rotational effects. Stresses were calculated along the vector that connected the first and last backbone atoms. The unfolding forces were applied in the opposite directions along this vector also, such as to increase the distance between the two atoms. Error in the force distributions of three molecules in the folded and unfolded states was estimated by the s.d. from the mean. We computed the error bar of each P ( F ) function measured over the entire trajectory by calculating this function from ten different independent shorter trajectories. The equilibrium part of the production trajectory was divided into ten equal parts and we then binned the P ( F ) from each. The s.d. of these P ( F ) from their mean was computed, and the resulting error bars are reported in Supplementary Figs S3-S8 . How to cite this article: Jose, P. P. & Andricioaei, I. Similarities between protein folding and granular jamming. Nat. Commun. 3:1161 doi: 10.1038/ncomms2177 (2012).